Contribution of the R-Ras2 GTP-binding protein to primary breast tumorigenesis and late-stage metastatic disease R-Ras2 is a transforming GTPase that shares downstream effectors with Ras subfamily proteins. However, little information exists about the function of this protein in tumorigenesis and its signalling overlap with classical Ras GTPases. Here we show, by combining loss- and gain-of-function studies in breast cancer cells, mammary epithelial cells and mouse models, that endogenous R-Ras2 has a role in both primary breast tumorigenesis and the late metastatic steps of cancer cells in the lung parenchyma. R-Ras2 drives tumorigenesis in a phosphatidylinostiol-3 kinase (PI3K)-dependent and signalling autonomous manner. By contrast, its prometastatic role requires other priming oncogenic signals and the engagement of several downstream elements. R-Ras2 function is required even in cancer cells exhibiting constitutive activation of classical Ras proteins, indicating that these GTPases are not functionally redundant. Our results also suggest that application of long-term R-Ras2 therapies will result in the development of compensatory mechanisms in breast tumours. R-Ras2 (also known as TC21) is a GTP-binding protein that, together with R-Ras1 and R-Ras3, forms part of the R-Ras GTPase subfamily [1] . This protein is the closest relative to classical Ras GTPases according to structural similarity criteria and, in fact, is the only Ras superfamily member that shows transforming activities similar to Ras oncoproteins [2] , [3] , [4] , [5] , [6] , [7] . Experiments using constitutively active versions of this protein revealed that R-Ras2 shares many Ras downstream signalling elements, including phosphatidylinostiol-3 kinases (PI3Ks) [7] , [8] , [9] , [10] , the Ral GDP dissociation stimulator (GDS) [7] , [11] and, in a cell type-specific manner, Raf kinases [4] , [5] , [6] , [12] , [13] . These properties led to the initial idea that this GTPase could represent an alternative avenue to stimulate the Ras pathway in tumours. In this context, R-Ras2 was considered as potentially important for breast tumorigenesis based on its frequent overexpression in human cancer cell lines and, in addition, its ability to drive transformation when expressed in immortalized breast cells [14] , [15] , [16] , [17] . Despite this, the interest on this GTPase faded away subsequently due to the absence of oncogenic RRAS2 gene mutations in tumours. However, recent reports have revived the interest on this protein in mammary gland-related processes. Thus, the analysis of Rras2 −/− mice has revealed that this GTPase plays proactive roles during mammary gland development [18] . Furthermore, recent observations have indicated that R-RAS2 could contribute to tamoxifen resistance [19] , [20] , thus suggesting that the inactivation of this pathway could be beneficial for patients with oestrogen receptor-positive breast tumours. It should be noted, however, that the systemic loss of R-Ras2 leads to unexpected protumorigenic effects in the case of mouse neurofibroma [21] that, if reproduced in other cancer types and in humans, may limit the interest of anti-R-Ras2-based therapies. Unfortunately, no information exists about the pros and cons of inactivating endogenous R-Ras2 in breast cancer in vivo and, therefore, about the actual therapeutic interest of this signalling route. Furthermore, as most of the work done with R-Ras2 has been based on the use of constitutively active versions and ectopic systems, we still have very few clues about the actual role of the endogenous protein and its functional redundancy with classical Ras GTPases. For the reasons stated above, we decided to revisit the function of R-Ras2 in different breast tumour subtypes using a comprehensive collection of genetic, signalling and animal model experiments. In the present study, we show that R-Ras2 has a role in the primary tumorigenesis and late metastatic steps of breast cancer cells. Such functions are required even when cancer cells have constitutive activation of classical Ras GTPases. Moreover, we show that the specific contribution of R-Ras2 to the overall transformation process is highly dependent on the cell type and malignant trait analysed. Our results also indicate that R-Ras2-based therapies will probably result in tumour recurrence through activation of signalling compensatory mechanisms. R-Ras2 affects primary tumorigenesis of breast cancer cells To evaluate the role of endogenous R-Ras2 in breast cancer and its redundancy with classical Ras proteins, we first used short hairpin RNA (shRNA) techniques to knock down the endogenous transcripts of this GTPase in both human MDA-MB-231-Luc and mouse 4T1 breast cancer cells. These cells represent good tools to address functional redundancy issues, because they exhibit constitutive activation of classical Ras proteins due to the presence of either oncogenic mutations (MDA-MB-231-Luc cells) [22] , [23] or autocrine signalling loops (4T1 cells) [24] . These cell lines also differ in metastatic potential, thus facilitating the use of both gain- and loss-of-function approaches to analyse the role of R-Ras2 in this process [25] . To rule out spurious effects derived from the cell-selection process, we used independent cell pools (labelled as ‘p1’ and ‘p2’) and clones (labelled as ‘c1’, ‘c2’ and ‘c3’) in these experiments. In addition, we used ‘rescued’ knockdown cell lines expressing a haemagglutinin (HA)-tagged version of human R-RAS2. When appropriate, we used cell line derivatives expressing a constitutively active version (G23V mutant) of HA-R-RAS2. A summary of all the MDA-MB-231-Luc and 4T1 cell lines used in this study can be found in Supplementary Tables 1 and 2 , respectively. Effective elimination or ectopic expression of indicated R-Ras2 proteins was verified by immunoblot analyses ( Supplementary Fig. 1 ). We observed that all MDA-M-231-Luc (KD RRAS2 .p1 and KD RRAS2 .p2; Fig. 1a–d ) and 4T1 (KD Rras2 .p1, KD Rras2 .c1, KD Rras2 .c2 and KD Rras2 .c3; Fig. 1e,f ) knockdown cells exhibited very low tumorigenicity when transplanted orthotopically in recipient mice. This was not due to off-target shRNA effects, because the expression of wild-type R-RAS2 ( Supplementary Fig. 1b,d ) rescued the in vivo tumorigenicity of both MDA-MB-231-Luc ( Fig. 1c,d ; see KD RRAS2 .p1+R-RAS2 cell line) and 4T1 ( Fig. 1f , bottom graph; see KD Rras2 .c1+R-RAS2 cell line) knockdown cells. The slow growth kinetics of tumours derived from R-Ras2-depleted cells were due to low proliferative and neoangiogenic rates rather than to enhanced apoptosis ( Supplementary Fig. 2 ). These results indicate that R-Ras2 is important for breast tumorigenesis even under constitutive Ras signalling conditions. Consistent with this lack of functional redundancy, we also observed that the ectopic expression of HA-R-RAS2 G23V further increased the in vivo tumorigenicity of K-RAS G13D - and B-RAF G464V -positive MDA-MB-231-Luc cells ( Fig. 1c,d ; see MDA+R-RAS2 G23V cells). This was associated with higher proliferative and angiogenic rates in tumours during their exponential growth phase ( Supplementary Fig. 2d,e ). These features were lost at later stages ( Supplementary Fig. 2a,b ), probably as a result of the very large size achieved by the tumour mass at that time (see above, Fig. 1c,d ). 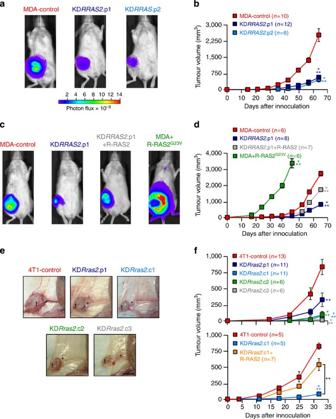Figure 1: R-Ras2 plays roles in primary tumorigenesis. (a) Example of a primary tumorigenesis experiment with indicated orthotopically transplanted MDA-MB-231-Luc cells. Scale of bioluminescence signals obtained in tumour-bearing animals is shown at the bottom. (b) Growth kinetics of tumours formed by indicated MDA-MB-231-Luc cells. ***P≤0.001 relative to values obtained by control cells at final experimental time point (number of independent transplants is indicated in the figure);t-test. (c) Example of a primary tumorigenesis experiment with indicated MDA-MB-231-Luc cells. (d) Growth kinetics of tumours formed by indicated MDA-MB-231-Luc cells. ***P≤0.001 relative to values obtained by control cells at the final experimental time point (number of independent transplants is indicated in the figure);t-test. (e) Example of tumours formed by indicated 4T1 cells. t, tumour; *, lymph node. (f) Growth kinetics of tumours formed by indicated 4T1 cells. **P≤0.01; ***P≤0.001 relative to values obtained by either control cells or indicated experimental pairs (in brackets) at final experimental time point (number of independent transplants is indicated in the figure);t-test. In panelsb,dandf, experimental values are given as mean± s.e.m. Figure 1: R-Ras2 plays roles in primary tumorigenesis. ( a ) Example of a primary tumorigenesis experiment with indicated orthotopically transplanted MDA-MB-231-Luc cells. Scale of bioluminescence signals obtained in tumour-bearing animals is shown at the bottom. ( b ) Growth kinetics of tumours formed by indicated MDA-MB-231-Luc cells. *** P ≤0.001 relative to values obtained by control cells at final experimental time point (number of independent transplants is indicated in the figure); t- test. ( c ) Example of a primary tumorigenesis experiment with indicated MDA-MB-231-Luc cells. ( d ) Growth kinetics of tumours formed by indicated MDA-MB-231-Luc cells. *** P ≤0.001 relative to values obtained by control cells at the final experimental time point (number of independent transplants is indicated in the figure); t- test. ( e ) Example of tumours formed by indicated 4T1 cells. t, tumour; *, lymph node. ( f ) Growth kinetics of tumours formed by indicated 4T1 cells. ** P ≤0.01; *** P ≤0.001 relative to values obtained by either control cells or indicated experimental pairs (in brackets) at final experimental time point (number of independent transplants is indicated in the figure); t- test. In panels b , d and f , experimental values are given as mean± s.e.m. Full size image R-Ras2 is involved in late metastatic steps As 4T1 cells are highly metastatic, we also examined the presence of metastasis in tumour-bearing animals at the end of the experiments shown in Fig. 1 . We observed that mice orthotopically transplanted with Rras2 -knockdown 4T1 cells seldom showed metastatic nodules in their lungs ( Table 1 ). This was not due to the lower growth rates of these tumours, because Rras2 -knockdown 4T1 cells could not form metastasis in the lung even when intravenously injected in mice ( Fig. 2a–c ). The metastatic defects shown by Rras2- knockdown cells in these two experimental systems were eliminated on expression of wild-type R-RAS2 in them ( Table 1 and Fig. 2b,c ). We also observed that ectopic R-RAS2 G23V enhanced the metastatic properties of parental 4T1 cells ( Fig. 2d,e and Supplementary Fig. 1d ; see 4T1+R-RAS2 G23V ). Even most notably, it triggered the acquisition of metastatic properties in the otherwise non-metastatic MDA-MB-231-Luc cell line ( Table 1 ; Fig. 2f ). Table 1 Metastasis formed by indicated 4T1 and MDA-MB-231-Luc cell lines in the lung and spleen on orthotopic transplantation in mammary pads. 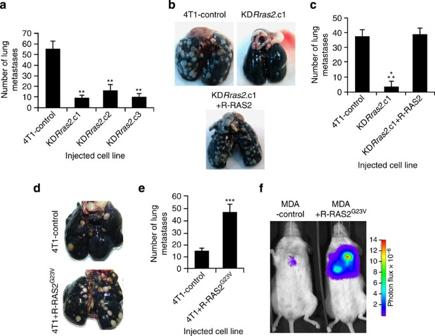Figure 2: R-Ras2 is important for breast cancer cell metastasis. (a) Lung metastases formed by indicated intravenously injected 4T1 cells. **P≤0.01 relative to control cell line (n=6, 12, 5 and 6 for 4T1-Control, KDRras2.c1, KDRras2.c2 and KDRras2.c3 cells, respectively);t-test. (b) Example of metastatic nodules (white spots) formed in lungs on intravenous injection of indicated 4T1 cells. (c) Lung metastases formed by indicated intravenously injected 4T1 cells. ***P≤0.001 relative to control cells (n=4, 5 and 6 for 4T1-Control, KDRras2.c1 and KDRras2.c1+R-RAS2 cells, respectively);t-test. (d) Examples of lung metastatic nodules formed by indicated intravenously injected 4T1 cell lines. (e) Lung metastases formed by indicated intravenously injected 4T1 cells. ***P≤0.001 relative to control cells (n=5). In this experiment, we injected suboptimal (5 × 104) numbers of 4T1 cells to pick up differences in metastatic node formation. (f) Example of lung metastatic behaviour of indicated intravenously injected MDA-MB-231-Luc cells (n=6). In panelsa,cande, experimental values are given as mean±s.e.m. Full size table Figure 2: R-Ras2 is important for breast cancer cell metastasis. ( a ) Lung metastases formed by indicated intravenously injected 4T1 cells. ** P ≤0.01 relative to control cell line ( n =6, 12, 5 and 6 for 4T1-Control, KD Rras2 .c1, KD Rras2 .c2 and KD Rras2 .c3 cells, respectively); t -test. ( b ) Example of metastatic nodules (white spots) formed in lungs on intravenous injection of indicated 4T1 cells. ( c ) Lung metastases formed by indicated intravenously injected 4T1 cells. *** P ≤0.001 relative to control cells ( n =4, 5 and 6 for 4T1-Control, KD Rras2 .c1 and KD Rras2 .c1+R-RAS2 cells, respectively); t -test. ( d ) Examples of lung metastatic nodules formed by indicated intravenously injected 4T1 cell lines. ( e ) Lung metastases formed by indicated intravenously injected 4T1 cells. *** P ≤0.001 relative to control cells ( n =5). In this experiment, we injected suboptimal (5 × 10 4 ) numbers of 4T1 cells to pick up differences in metastatic node formation. ( f ) Example of lung metastatic behaviour of indicated intravenously injected MDA-MB-231-Luc cells ( n =6). In panels a , c and e , experimental values are given as mean±s.e.m. Full size image The metastatic process involves a large number of steps, including lymph node infiltration, intravasation, extravasation and the subsequent survival and expansion of cancer cells in peripheral niches [26] , [27] . Using a quantitative reverse transcriptase–PCR (qRT–PCR) approach to quantify the presence of cancer cells in tissues, we observed that R-Ras2 was not required for the intravasation or lymph node dissemination of 4T1 cells ( Supplementary Fig. 3a ). We also observed that intravenously injected Rras2 -knockdown cells infiltrated the lung parenchyma at rates similar to control cells ( Supplementary Fig. 3b,c ), thus ruling out its implication in the extravasation process. To investigate its involvement in the post-extravasation phase, we analysed the effect of ectopic R-RAS G23V in mouse breast cancer cells that had specific defects in either the pre-extravasation (168FARN cells) or post-extravasation (4TO7 cells) steps ( Supplementary Fig. 3d,e ) [24] . Although inducing similar protumorigenic effects in these two lines ( Supplementary Fig. 3f ), we observed that R-RAS2 G23V could restore metastatic properties when expressed in 4TO7 but not in 168FARN cells ( Supplementary Fig. 3g–i ). These results indicate that the function of R-Ras2 in the metastatic process is circumscribed to the post-extravasation phase. R-Ras2 activates PI3K even in KRAS -transformed cells To understand the reason for the non-redundant role of R-Ras2 and Ras proteins in breast cancer cells, we next investigated the activation status of the downstream Erk, Akt and Ral-a signalling pathways in our collection of breast cancer cell lines. Consistent with the chronic activation of Ras proteins, we observed that control MDA-MB-231-Luc ( Fig. 3a ; top panel, compare lanes 1 and 5) and 4T1 ( Supplementary Fig. 4a ; top panel, compare lanes 1 and 5; Supplementary Fig. 4b , top panel, compare lanes 1 and 7) cells exhibited high amounts of phosphorylated Erk even under serum starvation conditions. Same results were obtained with 168FARN cells ( Supplementary Fig. 4b , upper panel, compare lanes 5 and 11). By contrast, 4TO7 cells showed serum-dependent Erk phosphorylation ( Supplementary Fig. 4b ; upper panel, compare lanes 3 and 9). All these cells unexpectedly showed serum-dependent phosphorylation of Akt ( Fig. 3a and Supplementary Fig. 4a ; third and fourth panels from top), indicating that the stimulation of this pathway was not directly linked to Ras activation status. These analyses also revealed that ectopic R-RAS2 G23V promoted a marked hyperphosphorylation of Akt in all cell lines tested. This effect was still serum-dependent in the case of 4T1 ( Supplementary Fig. 4a , third and fourth panel from top, compare lanes 4 and 8) and 4TO7 ( Supplementary Fig. 4b , third and fourth panels from top, compare lanes 4 and 10) cells, suggesting that R-RAS2 G23V is still subjected to some kind of upstream regulation in these cell lines. The stimulation of this signalling branch was specific, because R-RAS2 G23V did not induce any significant change in either Erk1/2 phosphorylation ( Fig. 3a and Supplementary Fig. 4a,b ; top panels) or Ral-a activity ( Supplementary Fig. 4c ). Hence, these results indicate that R-RAS2 G23V contributes to the stimulation of the PI3K/Akt route even in breast cancer cells with constitutive activation of classical Ras proteins. Consistent with this, we observed that ectopic R-RAS2 G23V also regulated a large number of Akt downstream elements ( Supplementary Fig. 4d–g ). Overexpressed wild-type R-RAS2 also elicited a mild, serum-dependent elevation in the amount of Akt phosphorylation in the ‘rescued’ knockdown cells ( Fig. 3a and Supplementary Fig. 4a ; third and fourth panels from top, compare lanes 1 and 3, and lanes 5 and 7). The use of PI3K isoform-specific inhibitors revealed that the activation of Akt by R-RAS2 G23V was mainly mediated by PI3Kα in both MDA-MB-231-Luc ( Fig. 3b ) and 4T1 ( Supplementary Fig. 4h ) cells. 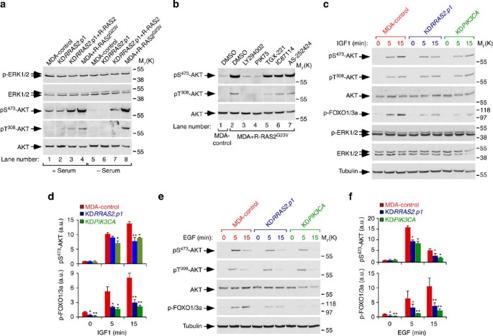Figure 3: Ectopic R-RAS2G23Vand endogenous R-RAS regulate the PI3Kα/AKT route in MDA-MB-231-Luc cells. (a) Phosphorylation and expression status of ERK and AKT proteins (left) in indicated MDA-MB-231-Luc cells (top) under exponentially growing (+ Serum) and serum-free (– Serum) conditions. p, phosphorylated. (b) Akt phosphorylation in indicated serum-starved MDA-MB-231-Luc cells (bottom) treated with PI3K family (LY294002, 20 μM), PI3Kα (PIK-75, 1 μM), PI3Kβ (TGX-221, 0.5 μM), PI3Kδ (IC-87114, 5 μM) and PI3Kγ (AS-252424, 0.5 μM) inhibitors (top). (c) Phosphorylation kinetics of AKT and FOXO1/3a in indicated, IGF1-stimulated MDA-MB-231-Luc cells. (d) Quantitation of phosphorylation kinetics of indicated proteins in above experiments (n=3). *P≤0.05; **P≤0.01 relative to values obtained in non-stimulated cells (which were given an arbitrary value of 1);t-test. (e) Phosphorylation kinetics of AKT and FOXO1/3a in indicated, EGF-stimulated MDA-MB-231-Luc cells. (f) Quantitation of phosphorylation kinetics of indicated proteins in above experiments (n=3). *P≤0.05; **P≤0.01 relative to values obtained in non-stimulated cells (which were given an arbitrary value of 1);t-test. In panelsdandf, experimental values are given as mean±s.e.m. Figure 3: Ectopic R-RAS2 G23V and endogenous R-RAS regulate the PI3Kα/AKT route in MDA-MB-231-Luc cells. ( a ) Phosphorylation and expression status of ERK and AKT proteins (left) in indicated MDA-MB-231-Luc cells (top) under exponentially growing (+ Serum) and serum-free (– Serum) conditions. p, phosphorylated. ( b ) Akt phosphorylation in indicated serum-starved MDA-MB-231-Luc cells (bottom) treated with PI3K family (LY294002, 20 μM), PI3Kα (PIK-75, 1 μM), PI3Kβ (TGX-221, 0.5 μM), PI3Kδ (IC-87114, 5 μM) and PI3Kγ (AS-252424, 0.5 μM) inhibitors (top). ( c ) Phosphorylation kinetics of AKT and FOXO1/3a in indicated, IGF1-stimulated MDA-MB-231-Luc cells. ( d ) Quantitation of phosphorylation kinetics of indicated proteins in above experiments ( n =3). * P ≤0.05; ** P ≤0.01 relative to values obtained in non-stimulated cells (which were given an arbitrary value of 1); t -test. ( e ) Phosphorylation kinetics of AKT and FOXO1/3a in indicated, EGF-stimulated MDA-MB-231-Luc cells. ( f ) Quantitation of phosphorylation kinetics of indicated proteins in above experiments ( n =3). * P ≤0.05; ** P ≤0.01 relative to values obtained in non-stimulated cells (which were given an arbitrary value of 1); t -test. In panels d and f , experimental values are given as mean±s.e.m. Full size image Unlike the above cases, we did not find any obvious alteration in the Akt signalling pathway in knockdown cells ( Fig. 3a and Supplementary Fig. 4a , compare lanes 1–2 and lanes 5–6). As this could be due to masking effects derived from the presence and absence of mitogens under the exponentially growing and serum-free culture conditions used, we decided to analyse the kinetics of activation of Akt on the stimulation of serum-starved RRAS2 -knockdown MDA-MB-231 cells with either insulin-like growth factor 1 (IGF1) or epidermal growth factor (EGF). These mitogens promote endogenous R-RAS2 activation, as demonstrated by pull-down experiments using a glutathione S -transferase–Ral GDS fusion protein that specifically recognizes GTP-bound R-RAS2 ( Supplementary Fig. 4i ) [11] . As a control for these experiments, we decided to use a stable MDA-MB-231-Luc cell line (referred to hereafter as KD PIK3CA ) in which the endogenous PIK3CA transcript was reduced ≈60% using shRNA techniques ( Supplementary Fig. 4j ). These cells showed no statistically significant variations in the relative amounts of PIK3CB and PIK3CG mRNAs when compared with controls ( n =3, P ≥0.05, t -test). However, they did show a small upregulation (1.85±0.09-fold) of PIK3CD transcripts (P ≤0.05, n =3, t -test). Using immunoblot analyses, we found that the depletion of endogenous R-RAS2 and PI3Kα reduced the IGF1- and EGF-mediated phosphorylation of AKT specifically in the mTORC2-dependent S 473 site ( Fig. 3c–f , compare first and second panels from top in each case). Such effect was more dramatic when the mitogen-triggered phosphorylation of FOXO1/3a was analysed in the same cell lysates ( Fig. 3c–f ). We also observed, using immunohistochemical techniques, that MDA-MB-231-Luc cell-derived tumours exhibited reduced phosphorylation levels of both FOXO1/3a and S6RP when compared with controls ( Supplementary Fig. 5 ). They also displayed increased immunoreactivity levels for p53 ( Supplementary Fig. 5 ), a tumour suppressor normally degraded through the PI3K/Akt/Mdm2 signalling axis ( Supplementary Fig. 4d ). Such defects were absent in tumours generated by ‘rescued’ RRAS2 -knockdown cells ( Supplementary Fig. 5 ). A tendency to a slight variation for the above markers was also observed in tumours generated by MDA+R-RAS2 G23V cells ( Supplementary Fig. 5 ). Taken together, these results indicate that R-Ras2 is important for the activation of a fraction of the PI3Kα present in KRAS -transformed breast cancer cells. R-Ras2 is important for protein translation in cancer cells MDA-MB-231 and 4T1 knockdown cells were unexpectedly quite similar to appropriate controls in terms of proliferative activity ( Supplementary Fig. 6a,b ), survival to anoikis ( Supplementary Fig. 6c,d ), the transcriptome ( Supplementary Fig. 6e ) and the proteome ( Supplementary Fig. 6f ; Supplementary Data 1 ). These results indicated that the alterations in tumour growth seen in vivo could not be due to intrinsic alterations in any of the above biological processes. This led us to analyse other potential R-Ras2 and PI3K/Akt/mTORC1-dependent routes that could contribute to the in vivo transforming properties of breast cancer cells. Consistent with the role of this signalling axis in protein synthesis regulation, we found that RRAS2- ( Fig. 4a,b ), Rras2 - ( Fig. 4c,d ) and PIK3CA- ( Fig. 4e,f ) knockdown cells, but not the ‘rescued’ knockdown cells ( Fig. 4e,f ), had less efficient protein synthesis than controls when tested using [ 35 S]-methionine labelling experiments. In agreement with the implication of the PI3K signalling pathway in this process, the ectopic expression of a constitutively active version of PI3Kα (PI3Kα CAAX mutant) [28] restored normal protein biosynthesis in MDA-MB-231-Luc knockdown cells ( Fig. 4e,f ; see KD RRAS2 .p1+PI3Kα CAAX cells). Corroborating these observations, we observed that all R-Ras2-deficient breast cancer cells had lower polysome over monosome percentages than controls ( Fig. 4g,h ). As above, such defect was not observed in knockdown cells expressing either PI3Kα CAAX ( Fig. 4g,h ) or wild-type R-RAS2 ( Fig. 4h ). Thus, in cell culture, endogenous R-Ras2 seems to contribute primarily to optimal protein biosynthesis in the two breast cancer cell lines under study. 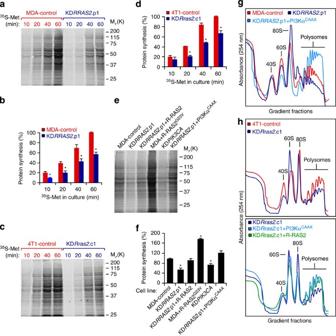Figure 4: R-Ras2 regulates protein translation in a PI3K-dependent manner. (a) Example of protein synthesis rates in indicated MDA-MB-231-Luc cells. (b) Quantitation of protein synthesis rates in indicated MDA-MB-231-Luc cells (n=3). *P≤0.05 relative to the control at each indicated time point;t-test. (c) Example of protein synthesis rates in indicated 4T1 cells. (d) Quantitation of protein synthesis rates in indicated 4T1 cells (n=3). *P≤0.05 relative to the control at each indicated time point;t-test. (e) Example of protein synthesis rates in indicated MDA-MB-231-Luc cells. (f) Quantitation of protein synthesis rates in indicated MDA-MB-231-Luc cells (n=3). *P≤0.05 relative to control cells;t-test. In panelsb,dandf, experimental values are given as mean±s.e.m. (g) Representative polysomal profiles of indicated MDA-MB-231-Luc cells (n=2). (h) Representative polysomal profiles of indicated 4T1 cells. Polysomal profiles obtained in the same experiment were split in two panels to facilitate the visualization of all lines. The KDRras2.c1-derived polysomal profile was included in both panels to facilitate the comparison of data presented (n=2). Figure 4: R-Ras2 regulates protein translation in a PI3K-dependent manner. ( a ) Example of protein synthesis rates in indicated MDA-MB-231-Luc cells. ( b ) Quantitation of protein synthesis rates in indicated MDA-MB-231-Luc cells ( n =3). * P ≤0.05 relative to the control at each indicated time point; t -test. ( c ) Example of protein synthesis rates in indicated 4T1 cells. ( d ) Quantitation of protein synthesis rates in indicated 4T1 cells ( n =3). * P ≤0.05 relative to the control at each indicated time point; t -test. ( e ) Example of protein synthesis rates in indicated MDA-MB-231-Luc cells. ( f ) Quantitation of protein synthesis rates in indicated MDA-MB-231-Luc cells ( n =3). * P ≤0.05 relative to control cells; t -test. In panels b , d and f , experimental values are given as mean±s.e.m. ( g ) Representative polysomal profiles of indicated MDA-MB-231-Luc cells ( n =2). ( h ) Representative polysomal profiles of indicated 4T1 cells. Polysomal profiles obtained in the same experiment were split in two panels to facilitate the visualization of all lines. The KD Rras2 .c1-derived polysomal profile was included in both panels to facilitate the comparison of data presented ( n =2). Full size image R-Ras2 promotes tumorigenesis in a PI3K-dependent manner Given the rescue effect elicited by PI3Kα CAAX in the above experiments, we next investigated whether the ectopic expression of this lipid kinase could also eliminate the in vivo defects exhibited by R-Ras2-depleted breast cancer cells. PI3Kα CAAX did restore the in vivo tumorigenicity of both knockdown cell lines ( Fig. 5a–d ) and, in the case of MDA-MB-231-Luc cells, promoted even higher tumorigenic activities than those normally shown by parental counterparts ( Fig. 5a,b ). The differential effect of PI3Kα CAAX in MDA-MB-231-Luc and 4T1 cells correlated well with the activation level of the PI3Kα/Akt signalling pathway achieved in each case ( Fig. 5e,f ). Confirming the involvement of PI3Kα in R-Ras2-dependent tumorigenesis, we observed that the partial knockdown of the endogenous PIK3CA transcript reduced the in vivo transforming activity of R-RAS G23V -expressing MDA-MB-231-Luc cells ( Fig. 5g,h , see MDA+R-RAS2 G23V +KD PIK3CA cells). However, these cells still formed tumours with growth kinetics similar to control cells, a result probably derived from the residual amounts of endogenous PI3Kα activity present in MDA+R-RAS2 G23V +KD PIK3CA cells ( Fig. 5e , compare lanes 1 and 5). The depletion of endogenous PI3Kα also reduced in vivo tumorigenic activity of parental cells ( Fig. 5a,b ). As in the case of the R-Ras2 depletion ( Supplementary Fig. 6a,b ), the in vivo tumorigenic defects shown by PI3Kα-deficient cells could not be attributed to reduced in vitro proliferation rates ( Fig. 5i ). 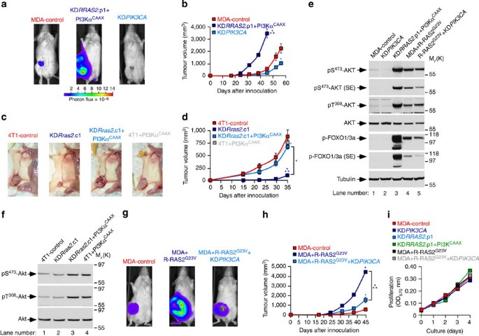Figure 5: The PI3Kα/Akt axis is important for R-Ras2-mediatedin vivotumorigenesis. (a) Representative example of tumours derived from indicated MDA-MB-231-Luc cells. (b) Growth rates of tumours derived from indicated MDA-MB-231-Luc cells (n=6). *P≤0.01; ***P≤0.001 relative to values obtained in control cells at final experimental time point;t-test. (c) Representative example of tumours formed by indicated 4T1 cells. (d) Growth rates of tumours derived from indicated 4T1 cells (n=6). *P≤0.01; ***P≤0.001 relative to values obtained in either control cells or the indicated experimental pairs (in brackets) at final experimental time point;t-test. (e) Phosphorylation and expression status of AKT and FOXO1/3a in indicated, serum-starved MDA-MB-231-Luc cells (top). A long (top panel) and short (SE, second panel from top) exposure is included for the anti-pS473AKT immunoblotting. (f) Phosphorylation and expression status of Akt in indicated, exponentially growing 4T1 cells. (g) Representative example of tumours formed by indicated MDA-MB-231-Luc cells (top). (h) Growth rates of tumours formed by indicated MDA-MB-231-Luc cells. *P≤0.01; ***P≤0.001 relative to values obtained in control cells or indicated experimental pairs (brackets) at final experimental time points (n=10, 10 and 4 for MDA-Control, MDA+R-RAS2G23Vand MDA+R-RAS2G23V+KDPIK3CA, respectively);t-test. (i)In vitroproliferation of indicated MDA-MB-231-Luc cell lines (n=3). In panelsb,d,handi, experimental values are given as mean±s.e.m. Figure 5: The PI3Kα/Akt axis is important for R-Ras2-mediated in vivo tumorigenesis. ( a ) Representative example of tumours derived from indicated MDA-MB-231-Luc cells. ( b ) Growth rates of tumours derived from indicated MDA-MB-231-Luc cells ( n =6). * P ≤0.01; *** P ≤0.001 relative to values obtained in control cells at final experimental time point; t -test. ( c ) Representative example of tumours formed by indicated 4T1 cells. ( d ) Growth rates of tumours derived from indicated 4T1 cells ( n =6). * P ≤0.01; *** P ≤0.001 relative to values obtained in either control cells or the indicated experimental pairs (in brackets) at final experimental time point; t -test. ( e ) Phosphorylation and expression status of AKT and FOXO1/3a in indicated, serum-starved MDA-MB-231-Luc cells (top). A long (top panel) and short (SE, second panel from top) exposure is included for the anti-pS 473 AKT immunoblotting. ( f ) Phosphorylation and expression status of Akt in indicated, exponentially growing 4T1 cells. ( g ) Representative example of tumours formed by indicated MDA-MB-231-Luc cells (top). ( h ) Growth rates of tumours formed by indicated MDA-MB-231-Luc cells. * P ≤0.01; *** P ≤0.001 relative to values obtained in control cells or indicated experimental pairs (brackets) at final experimental time points ( n =10, 10 and 4 for MDA-Control, MDA+R-RAS2 G23V and MDA+R-RAS2 G23V +KD PIK3CA , respectively); t -test. ( i ) In vitro proliferation of indicated MDA-MB-231-Luc cell lines ( n =3). In panels b , d , h and i , experimental values are given as mean±s.e.m. Full size image R-Ras2 uses different downstream effectors during metastasis Further analyses of tumour-bearing animals described in Fig. 5 revealed that PI3Kα CAAX contributed differently to the metastatic properties of 4T1 and MDA-MB-231-Luc cells. In the former case, ectopic PI3Kα CAAX could not restore the metastatic dissemination of Rras2 -knockdown 4T1 cells to the lung ( Table 2 ). This was not due to negative effects induced by this mutant protein, because PI3Kα CAAX did not impair the metastatic properties of parental cells ( Table 2 ). Similar results were found using intravenously injected cells ( Fig. 6a,b ). These results indicate that R-Ras2 is probably involved in two post-extravasation steps that are different according to PI3K signalling requirements. This additional signalling route entails hitherto unknown downstream elements, as our prior signalling data exclude the direct participation of the Raf/Erk and RalGDS/Ral-a axes in this process ( Fig. 3 and Supplementary Fig. 4a–c ). Consistent with this, we observed using rescue experiments with a number of R-RAS2 switch mutant versions [7] that the interaction with PI3K, but not with RalGDS, was important to maintain the R-Ras2-dependent metastatic phenotype of 4T1 cells ( Supplementary Fig. 7 ). In the case of MDA-MB-231-Luc cells, we observed that PI3Kα CAAX did trigger the acquisition of metastatic properties ( Table 2 ; Fig. 6c ). Conversely, the partial elimination of the endogenous PIK3CA transcript was sufficient to impair the metastatic phenotype induced by ectopic R-RAS2 G23V in these cells ( Table 2 ). These results indicate that R-Ras2 uses PI3Kα and other downstream elements to support metastatic traits in breast cancer cells (see Discussion). Table 2 Metastasis formed by indicated 4T1 and MDA-MB-231-Luc cell lines on orthotopic transplantation in mammary pads. 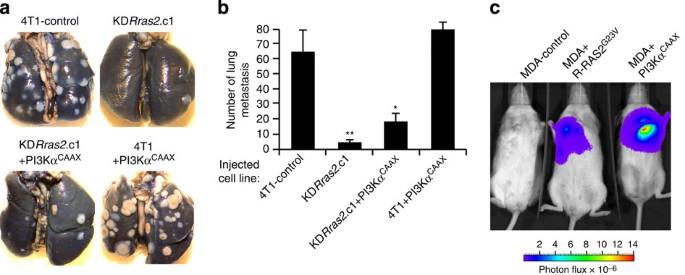Figure 6: R-Ras2 regulates late metastatic steps using PI3Kα-dependent and -independent mechanisms. (a) Example of metastatic nodules formed in lungs by indicated intravenously injected 4T1 cell lines. (b) Quantification of lung metastatic nodules formed by indicated intravenously injected 4T1 cell lines. Experimental values are given as mean±s.e.m. *P≤0.01; **P≤0.01 relative to control cells (n=4);t-test. (c) Metastatic colonization of lungs by indicated intravenously injected MDA-MB-231-Luc cells (n=4). The scale for the bioluminescence signal intensities recorded in these experiments is shown at the bottom. Full size table Figure 6: R-Ras2 regulates late metastatic steps using PI3Kα-dependent and -independent mechanisms. ( a ) Example of metastatic nodules formed in lungs by indicated intravenously injected 4T1 cell lines. ( b ) Quantification of lung metastatic nodules formed by indicated intravenously injected 4T1 cell lines. Experimental values are given as mean±s.e.m. * P ≤0.01; ** P ≤0.01 relative to control cells ( n =4); t -test. ( c ) Metastatic colonization of lungs by indicated intravenously injected MDA-MB-231-Luc cells ( n =4). The scale for the bioluminescence signal intensities recorded in these experiments is shown at the bottom. Full size image R-Ras2 promotes tumorigenesis in an autonomous manner To check the signalling autonomy of R-Ras2 in breast cancer initiation, we investigated the effect of ectopically expressing R-RAS2 G23V in primary mammary epithelial cells (MECs). The lentiviral-mediated expression of this protein in these cells ( Supplementary Fig. 8a ) led to the activation of the PI3K/Akt route ( Supplementary Fig. 8b ) and increased rates of PI3K-dependent proliferation ( Supplementary Fig. 8c–g ). This mitogenic effect was both serum- ( Supplementary Fig. 8d,e ) and Erk-independent ( Supplementary Fig. 8f,g ). In agreement with this, we did not see any upregulation of Erk proteins under these conditions ( Supplementary Fig. 8b ). Similar effects were seen with PI3Kα CAAX -expressing MECs ( Supplementary Fig. 8b,f,g ). On orthotopic transplantation, we observed that R-RAS2 G23V -expressing MECs generated glands with extensive ductal branching and very high numbers of terminal lobular-alveolar units ( Fig. 7a ). They also developed mammary tumours at high penetrance (six out of eight implanted samples) on very short latency periods ( Fig. 7b,c ). MECs infected with an empty lentivirus formed normal, non-tumorigenic mammary gland trees in recipient mice ( Fig. 7a ). Thus, these results indicate that R-Ras2-derived signals are sufficient to trigger the transformation of primary MECs both in vitro and in vivo . 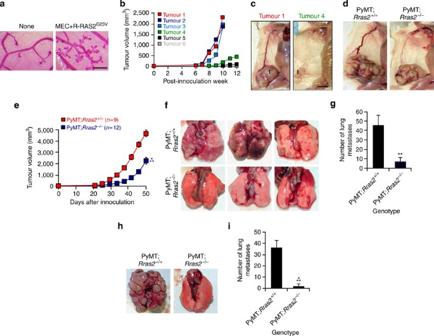Figure 7: R-RAS2G23Vpromotes transformation of primary MECs in a fully autonomous manner. (a) Example of histology of mammary glands generated 6 weeks after orthotopic implantation of control and HA-R-RAS2G23V-expressing MECs (n=4). Scale bar, 50 μm. (b) Growth kinetics of tumours induced by orthotopically transplanted HA-R-RAS2G23V-expressing MECs (n=8). (c) Example of tumours obtained in two of the recipient mice (numbers and colours are the same as those used inb. t, tumour. Scale bar, 1 cm. (d) Example of tumours formed by PyMT-infected MECs of indicated genotypes. (e) Growth kinetics of tumours formed by PyMT-infected MECs of indicated genotypes. ***P≤0.001 relative to control MECs (number of experiments is indicated in figure);t-test. (f) Example of lung metastases detected in animals bearing tumours from experiments shown indande. (g) Lung metastases detected in animals bearing tumours from above experiments. **P≤0.01 relative to control cells;t-test. (h) Example of metastatic nodules generated by intravenously injected tumour cells of indicated genotypes (top). (i) Quantification of lung metastatic nodules formed in experiments depicted inh. ***P≤0.001 relative to control MECs (n=5);t-test. Ine,gandi, values are given as mean±s.e.m. Figure 7: R-RAS2 G23V promotes transformation of primary MECs in a fully autonomous manner. ( a ) Example of histology of mammary glands generated 6 weeks after orthotopic implantation of control and HA-R-RAS2 G23V -expressing MECs ( n =4). Scale bar, 50 μm. ( b ) Growth kinetics of tumours induced by orthotopically transplanted HA-R-RAS2 G23V -expressing MECs ( n =8). ( c ) Example of tumours obtained in two of the recipient mice (numbers and colours are the same as those used in b . t, tumour. Scale bar, 1 cm. ( d ) Example of tumours formed by PyMT-infected MECs of indicated genotypes. ( e ) Growth kinetics of tumours formed by PyMT-infected MECs of indicated genotypes. *** P ≤0.001 relative to control MECs (number of experiments is indicated in figure); t -test. ( f ) Example of lung metastases detected in animals bearing tumours from experiments shown in d and e . ( g ) Lung metastases detected in animals bearing tumours from above experiments. ** P ≤0.01 relative to control cells; t -test. ( h ) Example of metastatic nodules generated by intravenously injected tumour cells of indicated genotypes (top). ( i ) Quantification of lung metastatic nodules formed in experiments depicted in h . *** P ≤0.001 relative to control MECs ( n =5); t -test. In e , g and i , values are given as mean±s.e.m. Full size image R-Ras2 promotes metastasis in a non-autonomous manner The examination of mice with breast tumours derived from implanted, R-RAS2 G23V -expressing MECs revealed no metastatic nodules or micrometastases in peripheral tissues, indicating that R-Ras2 was not fully autonomous to drive the de novo acquisition of metastatic traits. To distinguish if R-Ras2 did not play any metastasis-related role in primary cells or, alternatively, whether such role was subsidiary to the induction of metastatic traits by other oncogenic signals, we investigated the effect of the Rras2 gene deficiency in primary MECs transformed on the lentiviral-mediated expression of the polyoma middle T antigen (PyMT). Probably as a consequence of the PyMT-mediated activation of PI3Kα [29] , we observed that orthotopically transplanted PyMT + ; Rras2 −/− MECs could form tumours more efficiently than the immortalized breast cancer cells used in prior assays ( Fig. 7d,e ). Despite this, they still induced tumours at slightly lower kinetics than PyMT + ; Rras2 +/+ -transformed MECs ( Fig. 7d,e ). By contrast, the tumours generated by PyMT + ; Rras2 −/− MECs were conspicuously much less metastatic than those generated by the wild-type counterparts ( Fig. 7f,g ). The same metastatic defect was observed when cells isolated from those tumours were expanded in culture and injected intravenously in recipient mice ( Fig. 7h,i ). These observations indicate that R-Ras2 is required to maintain the metastatic phenotype triggered by other oncogenic signals rather than in the de novo induction of metastatic traits in primary cells. Endogenous R-Ras2 is important for Her2 tumorigenesis To assess the actual role of R-Ras2 in breast cancer under more physiological conditions, we finally used the mouse mammary tumour virus (MMTV)-Her2 tg mammary tumorigenesis model. In this transgenic system, the overexpression of the wild-type Her2 receptor (also known as Neu and Erbb2) in breast epithelial cells triggers mammary gland hyperplasia and, eventually, breast cancer. Thus, it recapitulates the transforming events that take place in human Her2 + breast tumours, a frequent PI3Kα/Akt-dependent breast cancer subtype [30] , [31] . To investigate the participation of R-Ras2 in this stepwise tumorigenic programme, we first analysed the structure of pre-neoplasic mammary glands in cohorts of pubertal MMTV-Her2 tg ; Rras2 +/+ and MMTV-Her2 tg ; Rras2 −/− female mice. This stage was selected because puberty is the period in which ducts undergo a major morphogenetic programme that eventually leads to the formation of the adult mammary gland [32] . At this stage, glands from MMTV-Her2 tg ; Rras2 −/− mice were smaller and less extended longitudinally than those from MMTV-Her2 tg ; Rras2 +/+ mice ( Fig. 8a,b ). In addition, they showed reduced numbers of terminal end buds (TEBs) ( Fig. 8a,b ), the structures responsible for duct bifurcation and elongation during this developmental period [32] . This phenotype is highly reminiscent of the developmental defects shown by single Rras2 −/− knockout mice at the same age [18] . In the post-pubertal period, glands from MMTV-Her2 tg ; Rras2 −/− mice were still slightly smaller ( Fig. 8a,b ) and lacked the extensive secondary and tertiary ductal branching typically observed at this developmental stage in glands from MMTV-Her2 tg mice ( Fig. 8a ), indicating that R-Ras2 is important for the premature lobulo-alveolar differentiation induced by overexpressed Her2 in post-pubertal mammary glands. This was a pathological-, Her2-specific function for R-Ras2, because mammary glands of Rras2 −/− mice do not show developmental defects at this stage [18] . To assess the status of PI3K and Erk in this system, we isolated MECs from prepubertal control and MMTV-Her2 tg ; Rras2 −/− mice and, on a short-term starvation period, stimulated them with EGF for the indicated periods of time. We observed that Rras2 -deficient MECs showed reduced Akt phosphorylation under these conditions. By contrast, the total amount and kinetics of Erk phosphorylation were not affected ( Fig. 8c ). 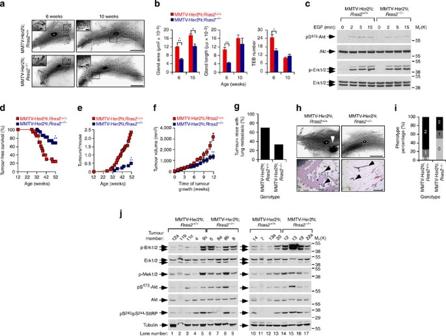Figure 8: R-Ras2 is important for Her2-mediated tumorigenesis. (a) Representative mammary fat pads from mice of indicated ages (top) and genotypes (left). Scale bar, 500 μm. Insets show enlarged views of boxed areas (scale bar, 50 μm). *Lymph node. (b) Quantification of area (left), maximal length (middle) and terminal end bud (TEB) numbers (right) of glands from mice of indicated ages and genotypes (n=5). *P≤0.05; **P≤0.01; ***P≤0.001 relative to appropriate control;t-test. (c) Phosphorylation and expression status of indicated proteins in EGF-stimulated MECs obtained from 6-month-old female mice. (d) Tumour-free survival of MMTV-Her2tg;Rras2+/+(n=20) and MMTV-Her2tg;Rras2−/−(n=22) mice. ***P≤0.001 relative to controls at the final experimental time point;t-test. (e) Tumour per mouse average in MMTV-Her2tg;Rras2+/+(n=20) and MMTV-Her2tg;Rras2−/−(n=22) mice. ***P≤0.001 relative to controls at the final experimental time point;t-test. (f) Average size of tumours developed in MMTV-Her2tg;Rras2+/+(n=20) and MMTV-Her2tg;Rras2−/−(n=22) mice. **P≤0.01 relative to controls at the final experimental time point;t-test. Inb,d,eandf, values are given as mean±s.e.m. (g) Mean percentage of tumour-bearing mice with lung metastases. (h) Representative whole mount-stained (top panels; scale bar, 500 μm) and haematoxylin/eosin-stained (bottom panels; scale bar, 100 μm) samples from inguinal, ‘non-tumorigenic’ mammary glands from indicated mice (top). White asterisks, inguinal lymph nodes; white arrowhead, example of a small adenocarcinoma; black asterisk, example of cystic dilation; black arrowheads, examples of hyperplasic lobulo-alveolar units. (i) Quantification of hyperplasic parameters in ‘non-tumorigenic’ mammary glands from indicated mice. Grade 0, no hyperplasia; grade 1, glands with ductal ramifications, lobulo-alveolar terminal units or cystic dilatations; grade 2, glands showing at least two of those hyperplasic parameters.n=15 and 21 control, and MMTV-Her2tg;Rras2−/−mice, respectively. (j) Phosphorylation and expression status of indicated proteins (left) in tumour samples (top) obtained from control and MMTV-Her2tg;Rras2−/−mice. Figure 8: R-Ras2 is important for Her2-mediated tumorigenesis. ( a ) Representative mammary fat pads from mice of indicated ages (top) and genotypes (left). Scale bar, 500 μm. Insets show enlarged views of boxed areas (scale bar, 50 μm). *Lymph node. ( b ) Quantification of area (left), maximal length (middle) and terminal end bud (TEB) numbers (right) of glands from mice of indicated ages and genotypes ( n =5). * P ≤0.05; ** P ≤0.01; *** P ≤0.001 relative to appropriate control; t -test. ( c ) Phosphorylation and expression status of indicated proteins in EGF-stimulated MECs obtained from 6-month-old female mice. ( d ) Tumour-free survival of MMTV-Her2 tg ; Rras2 +/+ ( n =20) and MMTV-Her2 tg ; Rras2 −/− ( n =22) mice. *** P ≤0.001 relative to controls at the final experimental time point; t -test. ( e ) Tumour per mouse average in MMTV-Her2 tg ; Rras2 +/+ ( n =20) and MMTV-Her2 tg ; Rras2 −/− ( n =22) mice. *** P ≤0.001 relative to controls at the final experimental time point; t -test. ( f ) Average size of tumours developed in MMTV-Her2 tg ; Rras2 +/+ ( n =20) and MMTV-Her2 tg ; Rras2 −/− ( n =22) mice. ** P ≤0.01 relative to controls at the final experimental time point; t -test. In b , d , e and f , values are given as mean±s.e.m. ( g ) Mean percentage of tumour-bearing mice with lung metastases. ( h ) Representative whole mount-stained (top panels; scale bar, 500 μm) and haematoxylin/eosin-stained (bottom panels; scale bar, 100 μm) samples from inguinal, ‘non-tumorigenic’ mammary glands from indicated mice (top). White asterisks, inguinal lymph nodes; white arrowhead, example of a small adenocarcinoma; black asterisk, example of cystic dilation; black arrowheads, examples of hyperplasic lobulo-alveolar units. ( i ) Quantification of hyperplasic parameters in ‘non-tumorigenic’ mammary glands from indicated mice. Grade 0, no hyperplasia; grade 1, glands with ductal ramifications, lobulo-alveolar terminal units or cystic dilatations; grade 2, glands showing at least two of those hyperplasic parameters. n =15 and 21 control, and MMTV-Her2 tg ; Rras2 −/− mice, respectively. ( j ) Phosphorylation and expression status of indicated proteins (left) in tumour samples (top) obtained from control and MMTV-Her2 tg ; Rras2 −/− mice. Full size image When analysed in long-term experiments, we found that MMTV-Her2 tg ; Rras2 −/− female mice developed mammary tumours at much lower frequencies than MMTV-Her2 tg ; Rras2 +/+ animals ( Fig. 8d ). When tumours developed, they required longer latencies ( Fig. 8d,e ), showed lower multiplicity ( Fig. 8e ) and were significantly smaller ( Fig. 8f ) and metastatic ( Fig. 8g ) than those from control mice. To assess the status of ‘non-tumorigenic’ glands, we isolated inguinal mammary glands from these cohorts of mice that, according to visual and palpation examination criteria, had not developed any physical sign of tumour outgrowth. Whole-mount and histological analyses revealed marked differences in the histology of these ‘non-tumorigenic’ glands. Thus, whereas a large percentage (≈70%) of inguinal glands from MMTV-Her2 tg ; Rras2 +/+ animals displayed extensive secondary ductal branching, increased numbers of lobulo-alveolar terminal units and cystic dilatation, the ‘non-tumorigenic’ ones from MMTV-Her2 tg ; Rras2 −/− animals only exhibited such hyperplasic phenotype in 30% of the cases examined ( Fig. 8h,i ). Taken together, these observations indicate that R-Ras2 plays important roles during Her2-induced mammary gland morphogenesis and tumorigenesis. R-Ras2 deficient tumours develop compensatory mechanisms Tumours from control and MMTV-Her2 tg ; Rras2 −/− mice were collected to analyse the phosphorylation and expression status of specific signalling routes typically involved in Ras and R-Ras2 transformation. Unexpectedly, we found using western blot analyses that seven out of the eight tumours obtained from MMTV-Her2 tg ; Rras2 −/− mice showed various levels of Erk1/2 hyperphosphorylation ( Fig. 8j , top panels, compare lanes 1–5/10–13 with 6–9/14–17). This was corroborated using immunohistochemical analyses with phospho-Erk1/2 antibodies ( Supplementary Fig. 9a ). Such upregulation was only observed in two out of the nine tumours obtained from control mice ( Fig. 8j , top panels; Supplementary Fig. 9a ). Further analysis indicated that Erk1/2 and Mek1/2 phosphorylation levels were usually, but not always co-regulated in the same tumour samples ( Fig. 8j , third panel from top). A more limited number of MMTV-Her2 tg ; Rras2 −/− mouse-derived tumours (50%) also showed increased amounts of phospho-Akt ( Fig. 8j , fourth panel from top). Elevated phosphorylation of S6RP was also observed in some of those tumours ( Fig. 8j , sixth panel from top). However, this event correlated better with the phospho-Erk rather than with the phospho-Akt status of those tumours ( Fig. 8j , compare first, fourth and sixth panels). Analysis of these tumours indicated that this compensatory mechanism was unrelated to the development of oncogenic mutations in Kras or Braf proto-oncogenes ( Supplementary Table 3 ) or to changes in expression of transcripts for either H-Ras or Erk phosphatases (Dusp1, Dusp2) ( Supplementary Fig. 9b ). We did observe cases of upregulation of the Kras mRNA in some of the samples analysed ( Supplementary Fig. 9b ). However, this parameter did not correlate with the amount of phospho-Erk found in the same tumour samples. The development of this signalling feature was not due to the direct activation of signalling crosstalk in pre-malignant stages, because MECs obtained from prepubertal MMTV-Her2 tg ; Rras2 −/− mice (see above, Fig. 8c ) and standard Rras2 −/− mice [18] do not show this signalling signature. R-Ras2 attracted significant interest on its discovery due to its high similarity to classical Ras GTPases. Despite this, we still have very little information about the actual role of endogenous R-Ras2 in tumours and the level of functional overlap with Ras proteins. To tackle those issues, we decided to use knockdown cancer cells, primary MECs and Rras2 −/− mice to assess the role of endogenous R-Ras2 in a number of breast cancer experimental models. In addition, we selected cancer cell lines that made it possible the direct examination of R-Ras2 function in the context of constitutive signalling from classical Ras GTPases. This multifaceted strategy revealed that endogenous R-Ras2 plays key functions during both primary breast tumorigenesis and late metastatic disease in the lung ( Supplementary Fig. 10 ). However, these roles change significantly depending on the cell background and signalling process analysed. For example, we have observed that R-Ras2 can drive primary tumorigenesis in a signalling autonomous manner. By contrast, it requires parallel signals from other oncogenic pathways to favour metastatic traits in both MECs and immortalized cancer cells ( Supplementary Fig. 10 ). The lack of functional autonomy of R-Ras2 in this latter process is probably a reflection of its specific involvement in post-extravasation metastatic stages, a feature that necessarily imposes the need of other oncogenic signals to favour the acquisition of earlier prometastatic traits such as efficient intravasation, survival behaviour in the circulation and extravasation properties. We have also found that R-Ras2 can drive primary tumorigenesis with (in the case of MECs) or without (in the case of immortalized cancer cells) parallel effects in mitogenic properties of cells, emphasizing the cell background-specific roles of this GTPase ( Supplementary Fig. 10 ). Our results have also unexpectedly revealed that R-Ras2 and classical Ras proteins work non-redundantly in breast cancer cells. We have demonstrated that part of such functional segregation involves the differential stimulation of the PI3Kα/Akt and Raf/Mek/Erk signalling axes by those proteins, respectively ( Supplementary Fig. 10 ). Although challenging the signalling dogma holding that the GTPase-dependent stimulation of PI3Kα is mostly mediated by direct physical interactions with oncogenic Ras proteins [33] , these results are consistent with previous data indicating that the PI3Kα/Akt axis can be activated in Ras-independent manners in some Ras-transformed cells [16] , [24] , [34] , [35] , [36] , [37] . Interestingly, the influence of R-Ras2 on the PI3K/Akt pathway is highly dependent on the experimental conditions used. Thus, we have seen that ectopically expressed R-RAS2 G23V promotes a marked upregulation of PI3K-dependent routes in all cell models analysed. By contrast, the depletion of the endogenous protein only affects the activation of a relatively small pool of the total PI3Kα present in breast cancer cells. As a consequence, we have observed that these cells only exhibit in vitro defects in protein biosynthesis, one of downstream responses regulated by the PI3K/Akt/mTORC route in cells. This is not entirely unexpected given that most cells can stimulate PI3Kα through different mechanisms, including the GTPase-independent physical interaction of PI3Kα/p85 PI3K complexes with upstream receptors [38] . Despite this, the R-Ras2-dependent PI3Kα pool is clearly relevant in vivo , given the marked tumorigenic and metastatic defects shown by R-Ras2-deficient breast cancer cells when implanted in recipient mice. The morphogenetic alterations seen in preneoplasic mammary glands of MMTV-Her2 tg ; Rras2 −/− mice, together with the signalling compensation events detected in tumours arising in those mice, are also indirect evidence in favour of defects in the PI3Kα/Akt/mTORC route in this experimental model [30] , [31] , [39] , [40] , [41] , [42] , [43] , [44] , [45] . However, as reconstitution experiments are not possible in this case, we cannot formally exclude the possibility that those events could be generated by defects in other R-Ras2-dependent signalling routes ( Supplementary Discussion ). Our results have revealed that R-Ras2 has to regulate other PI3Kα-independent signalling routes to maintain the metastatic properties of 4T1 cells ( Supplementary Fig. 10 ). This is consistent with recent observations indicating that full-blown metastasis in the lung parenchyma requires the coordinated and stepwise assembly of multiple biological programmes [46] . Unlike the case of 4T1 cells, we have observed that MDA-MB-231-Luc cells can acquire metastatic traits by just enforcing the stimulation of the PI3K/Akt axis through the expression of active versions of either R-RAS2 or PI3Kα. These two sets of results are not contradictory, as the rescue experiments performed in these two cell lines measure independent biological parameters. In the case of Rras2 -knockdown 4T1 cells, the ectopic expression of proteins is used to eliminate defects directly derived from the loss of endogenous R-Ras2 and, therefore, the results obtained can be directly used to infer the intrinsic signalling properties of R-Ras2 in the metastatic process. However, in the case of MDA-MB-231-Luc cells, the ectopic expression of proteins is used as a tool to elicit a gain-of-function effect in cells that have an R-Ras2 route intact. As a consequence, the rescue experiments give information in this case about the ability of R-RAS2 G23V and PI3Kα CAAX to overcome a PI3Kα-dependent (but R-RAS2-independent) post-extravasation step presumably defective in MDA-MB-231-Luc cells. Notwithstanding these results, the findings obtained in both experimental models clearly support the specific implication of PI3Kα as a key downstream element in the prometastatic signalling pathways of this GTPase. The results obtained with MMTV-Her2 tg mice further underscore the importance of endogenous R-Ras2 in breast tumorigenesis. This model also revealed that the lack of R-Ras2 promotes signalling compensation mechanisms in tumours similar to those seen before on the inactivation of specific PI3K/mTORC route signalling elements [39] , [40] , [41] , [42] , [43] , [44] , [45] . In those cases, such compensation effects are mostly mediated by the elimination of mTORC-dependent negative feedbacks on the Raf/Erk route [39] , [40] , [41] , [42] , [43] , [44] , [45] . However, the development of these signatures in MMTV-Her2 tg ; Rras2 −/− mice seems to require long-term Darwinian selection events, because primary MECs from both MMTV-Her2 tg ; Rras2 −/− (this work) and Rras2 −/− knockout mice [18] do not exhibit such signatures. Evidence for selection events favouring breast tumour recurrence do exist in the literature. Those include, for example, the amplification of Met , Erbb3 ( also known as Her3) , Myc and eiF4E genes [45] , [47] . It will be interesting to characterize the genome of Her2 tg ;Rras2 −/− tumours in the near future to verify whether they had developed similar or alternative genetic events during their outgrowth. An inference from these results is that R-Ras2-based therapies will probably fail in the long-term unless combined with drugs that could specifically block these signalling compensation events. Ethics statement All animal work has been done in accordance with protocols approved by the Bioethics committees of both the University of Salamanca and CSIC. Cell culture MDA-MB-231-Luc cells were provided by Dr. R. Gomis (Institute for Research in Biomedicine, Barcelona, Spain) and maintained in DulbeDMEM (Life Technologies) containing FCS (Life Technologies), 1% L -glutamine (Life Technologies) and 100 units ml −1 penicillin and streptomycin (Life Technologies). 4T1 cells were obtained from the ATCC and maintained as above in RPMI (Roswell Park Memorial Institute) media containing 10% FCS, penicillin (10 units ml −1 ) and streptomycin (100 μg ml −1 ). The 4OT7 and 168FARN cell lines were gently provided by Dr. F. Miller (Wayne State University School of Medicine, Detroit, MI) [25] and maintained as indicated for 4T1 cells. For cell stimulation studies, cancer cell lines were serum-starved for either 24 h (MDA-MB-231-Luc cells) or 4 h (4T1 cells), and then stimulated with EGF (20 ng ml −1 , Sigma) or IGF1 (50 ng ml −1 , Sigma) for the indicated periods of time. For the evaluation of the effect of PI3K inhibitors, serum-starved cells were incubated in serum-free media for 1 h with 20 μM LY294002 (Calbiochem), 1 μM PIK-75 (Cayman Chemical), 0.5 μM TGX-221 (Cayman Chemical), 5 μM IC-87114 (Cayman Chemical) or 0.5 μM AS-252424 (Cayman Chemical). Stock solutions for all those PI3K inhibitors were prepared in dimethylsulphoxide. According to the IC 50 values for each compound, PIK-75 must inhibit PI3Kα (IC 50 =5.8 nM) and, to a much lesser extent, PI3Kγ (IC 50 =0.076 μM) and PI3Kβ (IC 50 =1.3 μM) in experiments performed in this work. TGX-221 is regarded as a PI3Kβ-specific inhibitor [48] . IC-87114 must inhibit PI3Kδ (IC 50 =0.5 μM) while preserving the activity of both PI3Kγ (IC 50 =29 μM) and PI3Kβ (IC 50 =75 μM). According to previous data, this drug should not inhibit PI3Kα even if used at higher concentrations than those used in our in vivo experiments [49] . The AS-252424 compound must inhibit PI3Kγ (IC 50 =30 nM) and, to a much lesser extent, PI3Kα (IC 50 =0.94 μM). By contrast, it should not have significant effects on either PI3Kβ (IC 50 =20 μM) or PI3Kδ (IC 50 =20 μM). MECs were obtained from 8- to 12-week-old FVB mice. To this end, mammary glands 3, 4 and 5 were isolated, minced with a 22 scalpel for 3 min and digested in DMEM:F12 supplemented with 5% FCS, 2 mg ml −1 Clostridium histolyticum collagenase (Sigma), 100 μg ml −1 streptomycin, 100 units ml −1 penicillin) for 1 h at 37 °C under moderate shaking. Mammary organoids were separated from fat and single cells (such fibroblasts and red cells) by 600 g centrifugation steps lasting 10 min (one), 5 min (one), and 2 s (four). After each centrifugation step, cell pellets were resuspended in DMEM:F12 medium. Purified organoids were then trypsinized (0.5 mg ml −1 trypsin and 0.2 mg ml −1 EDTA in saline solution; Invitrogen) for 20 min at 37 °C, washed with DMEM:F12, incubated with DNAseI (4 units ml −1 in DMEM:F12, Sigma) for 3 min at 25 °C and filtered through a 70-μm cell strainer (BD Falcon). Cells were cultured in MEC primary growth medium (DMEM:F12 media containing 10% FCS, 5 μg ml −1 insulin, 5 ng ml −1 EGF (Sigma), 100 μg ml −1 streptomycin, 100 units ml −1 penicillin and 50 μg ml −1 gentamicin) from passages 0 to 2. For growth factor stimulation, MECs were incubated for 4 h in starvation medium (MEC primary growth medium lacking mitogens and containing 0.5% FCS) and then 5 nM EGF was added. To generate cultures from PyMT-induced breast tumours, a piece (≈1 cm 3 ) of the periphery of the tumour mass was dissected, minced with a 22 scalpel for 3 min and digested in DMEM:F12 supplemented with 5% FCS, 2 mg ml −1 Clostridium histolyticum collagenase (Sigma), 100 μg ml −1 streptomycin, 100 units ml −1 penicillin) for 1 h at 37 °C under moderate shaking. Cells were then spun down and trypsinized (0.5 mg ml −1 trypsin and 0.2 mg ml −1 EDTA in saline solution; Invitrogen) for 20 min at 37 °C, washed with DMEM:F12 (Invitrogen), and incubated with DNAseI (4 units ml −1 in DMEM:F12, Sigma) for 3 min at 25 °C. After being filtered through a 70-μm cell strainer (BD Biosciences/Falcon), cells were cultured in DMEM:F12 media containing 10% FCS, 5 μg ml −1 insulin, 5 ng ml −1 EGF, 100 mg ml −1 streptomycin, 100 units ml −1 penicillin and 50 μg ml −1 gentamicin) from passage 0 to passage 2. Western blot analyses Protein samples were separated electrophoretically and transferred onto nitrocellulose filters using the iBlot Dry Blotting System (Invitrogen). Membranes were blocked in either 5% non-fat dry milk (when immunoblotted with standard antibodies) or 5% BSA in (Sigma, when using phospho-specific antibodies) in TBS-T (25 mM Tris-HCl (pH 8.0), 150 mM NaCl, 0.1% Tween-20) for 1 h and then incubated overnight at 4 °C with appropriate primary antibodies (see Supplementary Table 4 ) diluted in blocking buffer. After three washes with TBS-T, the membrane was incubated with horseradish peroxidase-conjugated Protein A (Thermo Scientific) or the appropriate secondary antibody (Thermo Scientific, 1:5,000 dilution) for 1 h at room temperature. Immunoreacting bands were developed using a standard chemoluminescent method (Thermo Scientific). When indicated, films were scanned and immunoblot-derived signals quantified using the ImageJ software (National Institutes of Health). Full size images of blots are shown in Supplementary Figs. 11–17 . Animal studies For long-term tumorigenic experiments with cell lines, MDA-MB-231-Luc cells were trypsinized, resuspended in complete medium, counted, pelleted by centrifugation, washed once with ice-cold PBS, re-pelleted and resuspended (2 × 10 7 cell per ml) in a an ice-cold 50:50 solution of Matrigel (Growth Factor Reduced and Phenol Red-free; reference: 356231; BD Biosciences) and PBS. Fifty microlitres of the final cell suspension (1 × 10 6 cells) were introduced into the right inguinal mammary gland of anaesthetized, age-matched 4–6-week-old female NOD/SCID mice using a 25-gauge needle. 4T1 (usually 3,000 cells per implant, except in Supplementary Fig. 3f in which we used 500,000 cells per implant), 4TO7 (500,000 cells per implant) and 168FARN (500,000 cells per implant) were introduced in mammary fat pads as above. Tumour growth in each case was quantified by taking measurement of the tumour length ( L ), width ( W ) and depth ( D ). These parameters were then used to calculate the total tumour volumes at experimental time point using the mathematical formula: tumour volume= πLWD /6. Alternatively, tumour growth was assessed using as read-out the bioluminescence generated by the luciferase stably expressed by MDA-MB-231-Luc cells. To that end, orthotopically transplanted mice were injected intraperitoneally (150 μg g −1 of body weight) at the indicated time points with a D-luciferin (Promega) solution in PBS, anaesthetized with isofluorane and imaged using an IVIS system (Xenogen) coupled to Living Image Acquisition and Analysis software (Xenogen). Images were taken within the first 10 min after D-luciferin administration. Metastatic dissemination in tumour-bearing mice was quantified by both visually (in extracted lungs using a magnifying lens) and histologically (using tissue sections and standard light microscopy techniques) after killing the mice at the end of the in vivo tumorigenic experiments. To carry out direct, long-term lung colonization assays, 500,000 (50,000 in the case of Fig. 2d,e ) cells were resuspended in PBS as above and injected into the lateral tail vein. After 2 weeks, mice were euthanized, the chest cavity exposed through a midline chest incision, the trachea cannulated with a 20-gauge caterer and lungs slowly inflated using 1 ml of India ink (Parker, 1:16 dilution in PBS). Lungs were extracted, immersed in Fekete’s solution (100 ml 70% ethanol (Sigma), 10 ml 4% formaldehyde (Leica) and 5 ml 100% glacial acetic acid (Sigma)) to destain, and the metastatic nodules were counted by visual observation. Alternatively, lungs were extracted, fixed in 4% formaldehyde and embedded in paraffin for haematoxylin/eosin staining. Metastasis of MDA-MB-231-Luc cells were determined either by visual or bioluminiscence methods as above. In the case of assays with cancer cells derived from PyMT-expressing mammary tumours (see below), cells were resuspended in 100 ml PBS and injected (1 × 10 6 cells) into the tail vein of NOD/SCID female mice (Charles River) age-matched between 6 and 8 weeks. After 7 weeks, mice were euthanized, lungs extracted and metastatic nodules scored as above. To quantitate the dissemination of cancer cells to lymph nodes in tumour-bearing animals, we extracted total RNA from indicated lymph nodes using Trizol (Sigma) and the presence of circulating tumour cells indirectly estimated by qRT–PCR. This was done by calculating the abundance of the mRNA for the puromycin resistance gene (present exclusively in the 4T1 cells used in this study) in relation to that of an endogenous mouse mRNA ( B2m ). Primers used in these experiments are shown in Supplementary Table 5 . Values were corrected according to the expression of the viral gene in each cell line when maintained in tissue culture. To measure intravasation, we collected ≈1 ml of blood from the heart atrium of the same tumour-bearing mice, pelleted the circulating cells by centrifugation, lysed red cells using two lysis cycles in ACK buffer (BD Biosciences/Gibco) and extracted total RNAs using Trizol to quantify the presence of circulating tumour cells through qRT–PCR as above. To measure the extravasation of breast cancer cells, the indicated cell lines were labelled with 5 μM of a green cell tracker (CellTracker green CMFDA, Invitrogen) for 1 h and injected intravenously into mice (1 × 10 6 cells per mice). After 48 h, mice were injected intravenously with a rhodamine-conjugated lectin (Vector Laboratories) to stain lung capillaries and killed 60 min later. Lungs were then extracted, fixed in paraformaldehyde and examined by confocal fluorescence microscopy to visualize the number of cancer cells (green colour) present in the lung. For Her2-based tumorigenesis experiments, we crossed Rras2 −/− knockout [50] and MMTV-Her2 tg transgenic (FVB/NTg(MMTVneu)202 Mul/J strain; The Jackson Laboratory) mice to generate the compound MMTV-Her2 tg ; Rras2 mouse strain. The new strain was homogenized in the FVB background. For long-term tumorigenic experiments, mice were monitored for tumour development weekly as above. Experiments were finished when animals were 1 year old or, alternatively, when exhibiting either very large tumours or obvious signs of discomfort. At this time, the number of lung metastases was also determined visually as indicated above. In some cases, we also isolated mammary glands for histological examination that, according to palpation and visual examination, had not formed tumours during the above long-term tumorigenesis experiment. These glands indistinctly belonged to either tumour-free mice or to animals that had tumours in other mammary glands (that is, thoracic). These samples are referred to in main text as ‘non-tumorigenic’. Immunohistochemistry Depending on the experiment, the histology-related work was performed by independent personnel at the Histopathology units of either our Center or CNIO’s (Madrid, Spain). To this end, tissues were extracted, fixed in 4% paraformaldehyde (Sigma), cut in 2–3-μm-thick sections, and stained with haematoxylin/eosin. Proliferation and angiogenesis were monitored by immunohistochemical staining of tumour section with antibodies to Ki67 and CD31, respectively [18] , [51] . Apoptotic cells were detected using either TUNEL (TdT-mediated dUTP nick end labelling) labelling or cleaved caspase 3 immunostaining [18] . Additional immunohistochemical stainings were performed using a mouse monoclonal antibody to p53 (dilution 1:200; clone PAb 240, Abcam) and rabbit polyclonal antibodies to both phospho-T [24] FoxO1 and phospho-T [32] FoxO3a (dilution 1:10; catalogue number 9464, Cell Signaling Technology), phospho-S 240/244 S6RP (dilution 1:50; catalogue number 2215, Cell Signaling Technology) and phospho-Erk1/2 (dilution 1:400; catalogue number 9101, Cell Signaling Technology). For mammary gland development studies, mammary fat pads were extracted from animals of the indicated age, placed on dry, silanized glass slides and fixed overnight in Carnoy’s fixative (1:3:6 parts of glacial acetic acid:chloroform:100% ethanol). Tissues were rehydrated through successive incubations with 70% ethanol followed by distilled water and then stained with Red Carmine overnight. Mammary glands were analysed with a stereomicroscope (SMZ800, Nikon) and acquired with a digital camera (Digital Sight DS-Fi1, Nikon). The mammary gland area was obtained by calculating the area occupied by a lane drawn around the gland, including the nipple. The mammary gland length was measured from the end of the longest duct to a reference median point located between the nipple and the adjacent lymph node. In both cases, the analyses were carried out using ImageJ software (National Institutes of Health). Number of terminal end buds and branching points were counted using photomicrographs of the entire gland. Analysis of mRNA abundance Total RNAs were extracted using the RNeasy mini kit (Qiagen) and expression levels of transcripts determined by qRT–PCR using the QuantiTect SYBR Green RT–PCR kit (Qiagen) and a qRT–PCR apparatus (StepOnePlus Real-Time PCR System cycler, Applied Biosystems). Primers used for mRNA quantitation are described in Supplementary Table 5 . For normalization purposes, we measured in parallel the abundance of the endogenous transcript for human and mouse GAPDH ( Supplementary Table 5 ). Raw data were analysed using the StepOne software v2.1 (Applied Biosystems). In vitro proliferation and survival determinations We used the MTT (3-(4,5-dimethylthiazol-2-yl) 2,5-diphenyltetrazolium bromide) assay (Sigma) to determine the growth properties of cancer cells under study. To this end, cells were plated onto 24-well dishes (7,000 cells per well) and cultured in RPMI supplemented with 10% calf serum for the indicated periods of time. At the indicated time point, the culture medium of each well was discarded and replaced by 250 μl of an MTT solution (0.5 mg ml −1 ) in PBS. After 1 h at 37 °C in a 5% CO 2 atmosphere, 500 μl of dimethyl sulphoxide (Sigma) per well were added to dissolve the formazan crystals formed and the absorbance at the 570 nm wavelength measured 15 min later using a microplate reader (Ultraevolution, Tecan). In the case of MECs, aliquots of 20 × 10 3 MECs (passage 0–2, see above) were plated onto six-well culture plates and cultured in MEC primary growth medium. At the indicated time points, cells were trypsinized and counted. Alternatively, 5-bromodeoxyuridine incorporation assays were performed using a commercial kit (Cell Proliferation ELISA, Roche) according to the manufacturer’s instructions. To carry out three-dimensional culture studies, cells were trypsinized, washed, resuspended as a single-cell suspension in growth factor-reduced Matrigel and cultured in either starvation medium (MEC primary growth medium lacking mitogens and containing 0.5% FCS) or, alternatively, in standard MEC primary growth medium supplemented when needed with indicated drugs. After 10 days, bright-field pictures of cell colonies were acquired using an inverted microscope (Axiovert 135, Zeiss) coupled to a digital camera (C2724-95, Hamamatsu). After measuring the diameter ( D ) of the cell colonies using ImageJ software, the volume of colonies ( V ) was calculated using the following mathematical formula: V =4. π . ( D /2) 3 /3. When indicated, 0.2 μM wortmannin (Calbiochem) or 40 μM PD98059 (Calbiochem) were included in culture media. For cell survival determinations, cancer cells were seeded in either complete or serum-free media using both standard (at 25 × 10 4 cells per well) and ultra-low attachment surface six-well plates (5 × 10 5 cells per well) obtained from Corning. After either 24 h (in the case of 4T1 cells) or 48 h (in the case of MDA-MB-231-Luc cells), the percentage of viable cells was evaluated by flow cytometry using the Annexin V–fluorescein isothiocyanate apoptosis detection kit (Immunostep). Protein synthesis determinations Subconfluent, exponentially growing cells were maintained for 20 min in methionine-free DMEM (Life Technologies), washed once in PBS and re-cultured in methionine-free DMEM. After 20 min, cells were pulsed with 10 μCi of EasyTag L -[ 35 S]-Methionine (PerkinElmer). At the indicated periods of time, proteins were extracted using ice-cold lysis buffer (20 mM Tris-HCl (pH 7.4), 150 mM NaCl, 1% Nonidet-P40 (Sigma), 0.5% sodium deoxycholate (Sigma), 1 mM β-glycerophosphate (Sigma), 1 mM Na 3 VO 4 (Sigma), 50 mM NaF (Sigma) and a protease inhibitor cocktail (Cφmplete, Roche)), separated electrophoretically in 10% SDS–PAGE gels and transferred onto nitrocellulose filters using an iBlot Dry Blotting System (Invitrogen). After autoradiograph exposure of filters at −70 °C, the total amount of radiolabelled proteins was determined indirectly by densitometry analysis of autoradiography films using the ImageJ software. Polysome analyses were performed adapting a procedure previously described for Sachharomyces cerevisiae [52] . To this end, 6-8 × 10 7 cells were grown in 150 mm dishes to 80% confluency and, immediately before harvesting, treated with cycloheximide (0.1 mg ml −1 , Sigma) for 5 min at 37 °C. Cells were washed twice with ice-cold PBS containing 0.1 mg ml −1 cycloheximide and scraped off from plates using 2 ml of the same solution and a rubber policeman. Cells were collected by centrifugation and lysed by vortexing in 400 μl of polysome-profile lysis buffer (10 mM Tris-HCl (pH 7.5), 60 mM NaCl, 15 mM mgCl 2 , 0.5% Triton X-100 (Sigma), 0.1 mg ml −1 cycloheximide and 1 mg ml −1 heparine [Sigma]). After pre-clearing by high-speed centrifugation for 10 min at 4 °C, cell extracts equivalent to 5 absorption units at 260 nm were layered onto 7–50% sucrose gradients (10 ml), which had been prepared in 50 mM Tris-acetate (pH 7.5), 50 mM NaCl and 1 mM dithiothreitol. Ultracentrifugation was performed in a SW40 rotor (Beckman) at 39,000 r.p.m. for 165 min at 4 °C. Polysome profiles were obtained in a gradient reader apparatus (Brandel) by continuous reading of absorbance at 254 nm from the top to the bottom of each gradient. Genomic DNA sequencing Genomic DNA was extracted from samples of the mouse breast tumours shown in Fig. 8j using the QIAamp DNA micro kit (Qiagen) and sequences for Kras (exon 1) and Braf (exon 15) genes PCR amplified using appropriate oligonucleotides ( Supplementary Table 5 ). PCR products were sequenced at the Genomics and Proteomics Unit of our Center. Image processing Images were assembled and processed for final figure presentation using Canvas 9.0.4 (Deneba Systems). Statistics Statistical analyses were performed using the two-tailed Student’s t -test for paired and impaired data versus control values or, in other cases, the analysis of variance. Sample size was chosen to obtain statistically significant conclusions. No samples were excluded from analyses. With the exception of immunohistochemical data, score of experiments was not done blindly. Results with a P -value ≤0.05 were considered as statistically significant. Accession codes: The microarray data have been deposited in the Gene Expression Omnibus database under accession code GSE56615 . How to cite this article: Larive, R. M. et al. Contribution of the R-Ras2 GTP-binding protein to primary breast tumorigenesis and late-stage metastatic disease. Nat. Commun. 5:3881 doi: 10.1038/ncomms4881 (2014).